The oldest echinoderm faunas from Gondwana show that echinoderm body plan diversification was rapid The relatively sudden appearance of disparate animal lineages in the fossil record at the start of the Phanerozoic has been a focus of attention in palaeobiology ever since Darwin [1] first used this to argue for the incompleteness of the fossil record. While there is now no doubt about the reality of this event, both the underlying mechanisms and the duration and speed over which it took place remain matters of debate (for example, refs 2 , 3 , 4 ). A mixture of environmental, ecological and developmental drivers has been evoked to explain the appearance of complex animal life [3] , while the incomplete and patchy nature of the stratigraphical and fossil records from this time interval makes determining where and when clades arose problematic [4] . While early molecular clock approaches gave deep divergence dates for the origin of animal lineages (for example, ref. [5] 5) suggesting a massive failure of the fossil record, more recent approaches now provide a realistic and reliable time framework of events [6] , [7] . The origins of the great majority of phyla are now dated as late Cryogenian–Ediacaran in age (700–550 Ma). Nevertheless, this still points to substantial gaps in the fossil record, as the time between the inferred date of divergence (establishment of a lineage) and the first appearance of recognizable members of that lineage in the geological record can be substantial [8] . The record of the phylum Echinodermata exemplifies this perplexing pattern. Their fossil record starts in the early Cambrian (Series 2, Stage 3) with isolated plates. Articulated specimens first appear slightly later, in same stage, but they remain rare until the mid Cambrian (Series 3, late Stage 5) [9] . Initially, individual faunas typically contain just one dominant species, and have come almost exclusively from the palaeocontinent Laurentia. Later in the Cambrian, more diversified faunas make an appearance and echinoderms spread across diverse palaeogeographical regions of the world. Given that the rock record shows a gradual increase in diversity, it has been traditional to simply take this as an accurate record of echinoderm evolution (for example, refs 10 , 11 ). As these earliest echinoderm faunas comprise only ambulacral-bearing clades with radiate symmetry (helicoplacoids, stromatocystitids and gogiids), this has also been taken as evidence that the primitive echinoderm body plan was radiate and that asymmetric forms are derived (for example, refs 12 , 13 , 14 ). However, against this the most careful of molecular clock studies [7] , [15] place the divergence of echinoderms from their sister group, the hemichordates, in the late Ediacaran at ca. 570 Ma, implying some 50 my of missing echinoderm fossil record. Furthermore, some argue from comparative morphological grounds that peculiar asymmetric to bilaterally symmetric clades of echinoderm represent the primitive echinoderm body plan, even though they appear in the fossil record somewhat later than radiate forms [16] , [17] , [18] , [19] . While North America has the best representation of early Cambrian fossil echinoderms, new finds in the middle Cambrian (Series 3, late Stage 5) of Spain suggest that the echinoderm fossil record in Gondwana was both different and more diverse than in Laurentia [20] . Here, we report the discovery of new echinoderm faunas from Cambrian Stage 3 and from the Stage 4–5 boundary interval of Morocco, which represent the oldest faunas from Gondwana and are equivalent in age to the early Cambrian echinoderm-bearing strata in Laurentia. These faunas provide important new information on the variety of echinoderm body plans that existed in Gondwana at a time when the Laurentian record was very sparse. Geological setting and stratigraphy The Atlas Mountains of Morocco have extensive outcrops of Cambrian marine sediments that were laid down along West Gondwana ( Fig. 1 ). Early Cambrian sedimentation in Morocco began with the widespread development of subtropical shallow carbonate platforms dominated by Issendalenian microbial and archaeocyathan-microbial reefs (Igoudine and Amouslek formations [21] , [22] ). Subsequent tectonic rifting and block tilting in the Banian (Stages 3 and 4) resulted in a rapid drowning of successive rifting branches, in which deeper depressions (grabens and half-grabens) recorded the development of mud-mound complexes capped and surrounded by monotonous shales (Issafen Formation), whereas shallower environments recorded the development of dispersed archaeocyathan-microbial bioherms [23] , [24] . 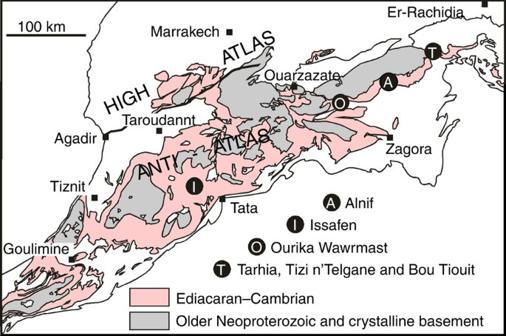Figure 1: Map of localities. Distribution of Cambrian rocks in Morocco and the location of the new fossil sites reported here. Figure 1: Map of localities. Distribution of Cambrian rocks in Morocco and the location of the new fossil sites reported here. Full size image The oldest of these offshore claystone-dominated facies, the Issafen Formation, crops out in the central Anti-Atlas ( Fig. 2 ). The formation at its type locality, east of the village of Timkit (Hupé [25] : pp. 64–67), is a transgressive shale-dominated unit, 100–180 m thick, with subsidiary nodular and bedded limestones and sandstones. Some rare decimetre-thick archaeocyathan-microbial biostromes and bioherms are present in the basal part, and contain archaeocyaths that correlate into the lower Botoman Substage of the Siberian Platform [26] , [27] . Above, the carbonate interbeds are dominated by bioclastic wackestones and packstones, and disarticulated echinoderm plates are common in both the shales and bioclastic limestones. At one level, first reported by Hupé [25] , complete echinoderm specimens occur within the Longianda and Gigantopygus Zones of the lower Tasousekhtian Substage [25] , [28] , subsequently correlated into the Antatlasia guttapluviae trilobite Zone of the middle Banian Substage [29] , global Stage 3. These are therefore the oldest echinoderms from Gondwana and the second oldest worldwide—only the Laurentian Poleta Formation of California with its fauna of helicoplacoids appears to be older. The lower part of the Issafen Formation at Lemdad Valley has been dated to 517 Ma by Maloof et al . [21] , but is highly diachronous throughout the Atlas Mountains, commencing in the Sectigena Zone of the late Banian in the southern High Atlas (Lemdad valley [27] , [30] ). 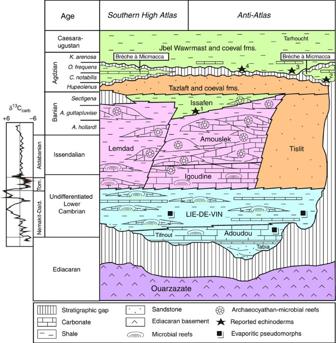Figure 2: Cambrian lithostratigraphy in Morocco. Summary lithofacies log showing how widespread shallow water microbial carbonates became replaced diachronously with offshore clastics during the Cambrian in Morocco. Chemostratigraphic data after Maloofet al.211, Issafen fauna; 2, Brèche à Micmacca Member fauna (Alnif, Tarhia); 3, basal Tarhoucht Member fauna (Tarhia, Tizi n'Telgane, Bou Tiouit); 4, Tarhoucht Member fauna (Jbel Wawrmast); Nemakit.-Dald, Nemakyt–Daldynian; Tom, Tommotian. Figure 2: Cambrian lithostratigraphy in Morocco. Summary lithofacies log showing how widespread shallow water microbial carbonates became replaced diachronously with offshore clastics during the Cambrian in Morocco. Chemostratigraphic data after Maloof et al . [21] 1, Issafen fauna; 2, Brèche à Micmacca Member fauna (Alnif, Tarhia); 3, basal Tarhoucht Member fauna (Tarhia, Tizi n'Telgane, Bou Tiouit); 4, Tarhoucht Member fauna (Jbel Wawrmast); Nemakit.-Dald, Nemakyt–Daldynian; Tom, Tommotian. Full size image Our second echinoderm-rich fossil assemblage of early Cambrian age from the Atlas Mountains is related to another transgression. In the eastern Anti-Atlas, the coarse, shallow-water sandstones of the Tazlaft Formation (lower Stage 4) are succeeded by a broad deepening of the whole platform and the onset of the fine siliciclastics of the Jbel Wawrmast Formation ( Fig. 2 ). These deposits commence with alternations of hiatal shell-volcaniclast accumulation layers capped with stromatolitic crusts and variegated claystones (Brèche à Micmacca Member [31] , [32] , [33] ). At two localities, one near Alnif and the other close to Tarhia ( Fig. 1 ), a claystone level close to the base of the member contains trilobites indicative of the base of the Cephalopyge notabilis Zone [29] . These offshore clastics thus date from the global Stage 4–5 boundary interval, and are approximately contemporary with the echinoderm-bearing Kinzers Formation of North America. Shell beds become episodic up section and eventually disappear. The upper claystone-dominated part of the Jbel Wawrmast Formation (the Tarhoucht Member) consists of offshore shales with occasional levels rich in trilobites and with articulated echinoderms. This level has been sampled at various localities in the eastern Anti-Atlas, including Tarhia, Tizi n'Telgane and Bou Tiouit. It contains trilobites typical of the ‘briareus beds’ ( sensu Geyer et al . [34] ) indicative of the upper part of the Cephalopyge notabilis Zone. Some of the echinoderms at this level are the same as those from the Brèche à Micmacca Member but not all, with the stylophoran Ceratocystis making its first appearance. A second and slightly younger level within the Tarhoucht Member was sampled at the Ourika Wawrmast stratotype. It lacks trilobites with the exception of some isolated sclerites making correlation difficult, but Geyer et al . [34] dated it as Ornamentaspis frequens Zone or Cephalopyge notabilis Zone and thus falling within global Stage 5. This level is important in terms of echinoderms because it lacks the previous mentioned fauna with the exception of pieces from edrioasteroids, but it contains two novel morphologies, the lichenoidid eocrinoid and the columnal-bearing eocrinoid. 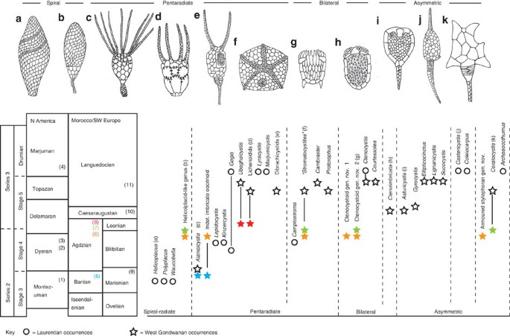Figure 3: Stratigraphic distribution of early to middle Cambrian echinoderms. Summary of the stratigraphic distribution of echinoderm fossils based on articulated specimens found in Laurentia (North America) and western Gondwana (France, Spain and Morocco). Strata with main fossil echinoderm faunas are numbered and are as follows: (1) Poleta Formation; (2) Latham Shale Formation; (3) Kinzers Formation; (4) Various Drumian-aged formations, including the Marjum Formation, and Burgess Shale Formation; (5) Issafen Formation; (6) Jbel Wawrmast Formation (Brèche à Micmacca Member); (7) Jbel Wawrmast Formation (Tarhoucht Member 1); (8) Jbel Wawrmast Formation (Tarhoucht Member 2); (9) ‘Alanís beds’; (10) Genestosa Member (Oville Formation) and Murero Formation (part); (11) Murero Formation (part) and Borobia Formation. Circles indicate genera from North America and stars indicate genera from West Gondwana. Coloured stars are new records from Morocco. Correlation between West Gondwana and North America follows Gradsteinet al.48 Cambrian echinoderm faunas Figure 3 summarizes the stratigraphic distribution of levels that have yielded articulated echinoderms from the early part of the Cambrian (Series 2 and 3) in Laurentia (North America) and western Gondwana (France, Spain and Morocco). It also summarizes the distribution of echinoderms from these regions, highlighting the new taxonomic discoveries from Morocco being reported here. Echinoderms are divided into four informal groups according to their body symmetry and possession of ambulacra; bilaterally symmetrical forms lacking ambulacra, asymmetric forms lack ambulacra or with a single ambulacrum, and spiral-radiate and pentaradiate forms having multiple ambulacra arranged radially around the mouth. The Issafen Formation ( Fig. 3 , level 5) has yielded the oldest articulated echinoderms from Gondwana and is dominated by a new species of the gogiid Alanisicystis. This has a short polymeric column, a single basal cup plate and sack-like polyplated body with triserial ambulacra giving rise to clusters of long straight brachioles ( Fig. 4d ). Alanisicystis has previously been recorded from Spain, close to the Stage 3–4 boundary [35] and is approximately equal in age to the earliest gogiid in North America, Gogia ojenai [36] , which differs most obviously in lacking a large basal cup plate. Also in the same bed at Issafen is a second species, a lepidocystid, closely similar to and possibly congeneric with Lepidocystis [37] ( Fig. 4k ). There is insufficient material as yet to determine its taxonomic status more accurately but our material shows the typical brachioles and the characteristic arrangement of large and small thecal plates across the oral surface of this genus. This is the first record of lepidocystids outside Laurentia and extends their range deeper into the early Cambrian. Figure 3: Stratigraphic distribution of early to middle Cambrian echinoderms. Summary of the stratigraphic distribution of echinoderm fossils based on articulated specimens found in Laurentia (North America) and western Gondwana (France, Spain and Morocco). Strata with main fossil echinoderm faunas are numbered and are as follows: (1) Poleta Formation; (2) Latham Shale Formation; (3) Kinzers Formation; (4) Various Drumian-aged formations, including the Marjum Formation, and Burgess Shale Formation; (5) Issafen Formation; (6) Jbel Wawrmast Formation (Brèche à Micmacca Member); (7) Jbel Wawrmast Formation (Tarhoucht Member 1); (8) Jbel Wawrmast Formation (Tarhoucht Member 2); (9) ‘Alanís beds’; (10) Genestosa Member (Oville Formation) and Murero Formation (part); (11) Murero Formation (part) and Borobia Formation. Circles indicate genera from North America and stars indicate genera from West Gondwana. Coloured stars are new records from Morocco. Correlation between West Gondwana and North America follows Gradstein et al . 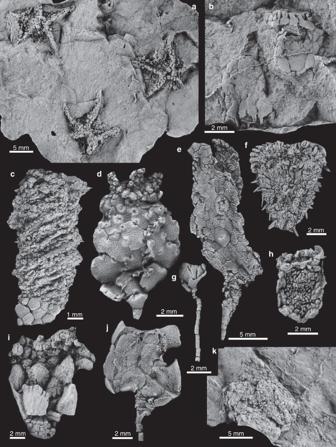Figure 4: Examples of echinoderms from the Cambrian Stages 3–5 of Morocco. (a)Stromatocystitessp. (stromatocystitid); Tarhoucht Member, Level 7, Stage 4–5 boundary interval. (b) Ctenocystoid gen. et sp. nov. 2; Tarhoucht Member, Level 7, Stage 4–5 boundary interval. (c) Helicoplacoid-like form, gen. et sp. nov.; Tarhoucht Member, Level 7, Stage 4–5 boundary interval. (d)Alanisicystissp. nov. (gogiid); Issafen Formation, Level 5, Stage 3. (e) armoured stylophoran gen. et sp. nov.; Brèche à Micmacca Member, Level 6, Stage 4–5 boundary interval. (f) Ctenocystoid gen. et sp. nov. 1; Brèche à Micmacca Member, Level 6, Stage 4–5 boundary interval, (g)Ubaghsicystissp. (columnal-bearing eocrinoid); Tarhoucht Member, Level 8, Stage 5. (h) Ctenocystoid gen. et sp. nov. 2; Brèche à Micmacca Member, Level 6, Stage 4–5 boundary interval. (i) Lichenoidid gen. et sp. nov.; Tarhoucht Member, Level 8, Stage 5. (j)Ceratocystis(armoured stylophoran); Tarhoucht Member, Level 7 Stage 4–5 boundary interval. (k) Lepidocystid cf.Lepidocystissp.; Issafen Formation, Level 5, Stage 3. [48] Full size image Figure 4: Examples of echinoderms from the Cambrian Stages 3–5 of Morocco. ( a ) Stromatocystites sp. (stromatocystitid); Tarhoucht Member, Level 7, Stage 4–5 boundary interval. ( b ) Ctenocystoid gen. et sp. nov. 2; Tarhoucht Member, Level 7, Stage 4–5 boundary interval. ( c ) Helicoplacoid-like form, gen. et sp. nov.; Tarhoucht Member, Level 7, Stage 4–5 boundary interval. ( d ) Alanisicystis sp. nov. (gogiid); Issafen Formation, Level 5, Stage 3. ( e ) armoured stylophoran gen. et sp. nov.; Brèche à Micmacca Member, Level 6, Stage 4–5 boundary interval. ( f ) Ctenocystoid gen. et sp. nov. 1; Brèche à Micmacca Member, Level 6, Stage 4–5 boundary interval, ( g ) Ubaghsicystis sp. (columnal-bearing eocrinoid); Tarhoucht Member, Level 8, Stage 5. ( h ) Ctenocystoid gen. et sp. nov. 2; Brèche à Micmacca Member, Level 6, Stage 4–5 boundary interval. ( i ) Lichenoidid gen. et sp. nov.; Tarhoucht Member, Level 8, Stage 5. ( j ) Ceratocystis (armoured stylophoran); Tarhoucht Member, Level 7 Stage 4–5 boundary interval. ( k ) Lepidocystid cf. Lepidocystis sp. ; Issafen Formation, Level 5, Stage 3. Full size image The earliest diverse echinoderm fauna appears in the Brèche à Micmacca Member of the Jbel Wawrmast Formation in the upper part of Stage 4 or base of Stage 5 at a level approximately equivalent to the Kinzers Formation of Laurentia ( Fig. 3 , level 6). Here representatives from five very different clades of echinoderm occur together, though never in great numbers. At this level pelmatozoans are rare, with only the occasional fragmentary remains of an imbricate eocrinoid with biserial brachioles present. The most commonly encountered forms are two new genera of ctenocystoid ( Fig. 4f ) and a new stromatocystitid close to Stromatocystites ( Fig. 4a ). One ctenocystoid ( Fig. 4f ) has near perfect bilateral symmetry, has a larger number of ossicles in its ctenidium, lacks any marginal frame and has circumferential bands of spinose plates. The second ( Fig. 4h ) is a more derived form that has a uniserial frame of marginal with a pair of posterior spines and fewer ctenoid plates. The stromatocystitid is represented by numerous individuals of various sizes, with the smallest showing a well-defined peripheral ring of plates. Before this, the oldest ctenocystoid and stromatocystitid came from the Murero Formation of Spain in beds that are late Stage 5 in age or Drumian [38] . Accompanying these is a primitive armoured stylophoran with a bipartite appendage and asymmetric body composed of a large number of small plates ( Fig. 4e ). The Brèche à Micmacca Member also contains a very interesting helicoplacoid-like echinoderm, which has a well-defined polymeric stalk and basal cup, topped by a spirally plated, cone-shaped body with apical mouth ( Fig. 4c ). While the cone-shaped body of this animal closely resembles the helicoplacoid Waucobella from Laurentia, both having spiral rows of thorn-like plates, its possession of a stalk and basal cup of thick plates like that of eocrinoids make it very different from any Laurentian helicoplacoid. This discovery resolves a long-standing problem concerning the homologies that exist between helicoplacoids and other echinoderms, and will transform how we view them phylogenetically. However, as this requires a detailed description of the taxon, something that is beyond the scope and aims of this paper, we leave this discussion to a subsequent paper. Slightly higher in the Jbel Wawrmast Formation, from Stage 5 ( Fig. 3 , level 7), articulated specimens of the armored stylophoran Ceratocystis ( Fig. 4j ) are found coexisting with several taxa from the underlying level. Isolated elements of this animal have previously been reported from the Brèche à Micmacca Member [39] but articulated specimens have so far only been recovered from level 7 (see Fig. 3 ). This represents the oldest recorded Ceratocystis that approximately matches in age a single specimen collected from Germany [40] . This level also contains a ctenocystoid closely similar to that seen in the earlier level ( Fig. 4b ). Two eocrinoids also appear in a slightly younger level but from a different locality ( Fig. 3 , level 8), a holomeric stemmed eocrinoid with a globular theca closely related to Ubaghsicystis ( Fig. 4g ) and a new genus of lichenoidid eocrinoid ( Fig. 4i ). This last form has brachioles that attach to horse shoe-shaped facets on the perioral plates, and has highly thickened and enlarged basal plates and a rudimentary stalk. Other taxa also occur, but are currently too poorly known to be placed with certainty. The Issafen Formation contains the oldest articulated fossil echinoderms from Gondwana, while the Brèche à Micmacca Member of the Jbel Wawrmast Formation has the earliest diverse echinoderm fauna worldwide. These new discoveries extend the ranges of several major clades (stylophorans, ctenocystoids, stromatocystitids and lychenoidid ‘eocrinoids’) back to the Stage 4–5 boundary interval where previously there were few records. Importantly this now highlights that almost from the start of their fossil record, echinoderms with four clearly differentiated body plans coexisted: pentaradiate forms (stromatocystitids and gogiids), asymmetric forms (ceratocystitid stylophorans), bilateral forms (ctenocystoids) and spiral forms (helicoplacoids). While the discovery of a new spirally plated taxon fills the gap between helicoplacoids and stalked echinoderms, the morphological gap between these ambulacral-bearing echinoderms and echinoderm groups lacking ambulacra remains striking. Furthermore, ctenocystoids and stylophorans are as highly differentiated from other clades at their first appearance as they are later in their fossil record. The appearance of articulated echinoderms in the fossil record of Gondwana is intimately associated with platform drowning in a rifting context and the appearance in the surviving rock record of the earliest extensive claystones deposited in offshore environments ( Fig. 2 ). This is true both in the central and eastern Anti-Atlas, where separate drowning events each saw the commencement of offshore lithofacies in the region and the simultaneous appearance of echinoderm faunas. Taken together with the morphological disparity encompassed by these earliest faunas, this implies that there is a strong palaeogeographical and/or palaeoenvironmental control to the early fossil record of echinoderms, with faunas tracking offshore facies. With such small time differences now separating the first occurrences of radiate, spiral, bilateral and asymmetric echinoderms, little significance should be placed on their stratigraphical order of appearance. Furthermore, it is likely that earlier stages of echinoderm evolution remain hidden because the stratigraphical record is so incomplete that it has failed to capture appropriate offshore claystone facies from the late Ediacaran–early Cambrian like those from which the first diverse faunas are recorded. What we see in West Gondwana is the stepwise immigration of an already diversified fauna as open marine conditions and microbial mat-free clayey substrates spread across the Moroccan rift following extensional tilting and it is this change in environmental representation that is shaping the fossil record. But just how much record is actually missing, and how rapidly did echinoderm body plans evolve? Molecular clock estimates such as those of Peterson et al . [6] , Erwin et al . [7] and Pisani et al . [15] place the origin of echinoderms in the late Precambrian, at around 570 Ma and several 10 s of millions of years before the first articulated specimens are found. However, this dates the origins of total group echinoderms, and identifying the most primitive members of any clade can be highly problematic simply because of the lack of diagnostic, fossilizable characters in those taxa [41] . However, echinoderms have a mineralized skeleton with a very distinctive morphology termed stereom that is underpinned by a unique family of genes [42] . It is the first synapomorphy of echinoderms that can be recognized [17] and the evolution of a mesoskeleton composed of stereom must thus predate diversification of the clade into bilateral, asymmetrical, spiral-radiate and pentaradiate body plans. Because of its distinctive microstructure, even isolated plates of echinoderms are easily recognizable in petrological thin sections. It is therefore noteworthy that the earliest ossicles showing stereom appear more or less contemporaneously in Siberia, Laurentia and Gondwana, within the Delgadella anabara Zone of Cambrian Series 2, Stage 3 (Atdabanian), at between 520 and 525 Ma [9] , [43] . Furthermore, no recognizable stereom plates have yet been discovered among the slightly earlier small shelly Tommotian faunas. While this just provides a latest date by which echinoderms acquired their stereom skeleton, the mineralogical composition of the skeleton also supports an origin of biomineralization in the early Cambrian. The calcium carbonate mineralogies utilized by organisms in constructing their skeletons have been shown to reflect fluctuations in the magnesium/calcium ratio of sea water that occurred from late Ediacaran to early Cambrian times [43] , [44] , [45] , [46] . Organisms with a calcium carbonate skeleton apparently utilized the polymorph that was most favourable with respect to ambient seawater conditions at the time, and that, once a clade evolved its skeleton, it usually retained that polymorph type for the remainder of its history [44] . Based on early marine precipitates and cements and fluid inclusion data, a major change in ocean geochemistry took place in the early Cambrian (within Stage 2 at around the Nemakit–Daldynian–Tommotian boundary), transforming oceans from aragonite to calcite seas. This change coincided with a major perturbation in the Carbon cycle that resulted in a 10% negative shift in δ 13 C 43 in ocean geochemistry, and may have been triggered by influx of continental weathering products during the last stages in the formation of the great unconformity in Laurentia [47] . Clades with aragonite skeletons mostly originate from before 525 Ma, while those with calcite skeletons largely post-date this event. Interestingly, clades with high-magnesium carbonate skeletons appear in the fossil record clustered around the transition from aragonite to calcite seas in the upper part of Stage 2 (Tommotian) corresponding to the transitional phase in ocean geochemistry of falling Mg/Ca ratio [43] . As echinoderms have a skeleton of high-magnesium calcite, his lends support to the view that echinoderms evolved biomineralization at around this time. Our discovery that echinoderms displaying several disparate body plans were already in existence by the end of Cambrian Stage 4, so soon after a major change in sea-water chemistry and the appearance of stereom plates in the fossil record, is a critical discovery. Either stereom was independently acquired (which seems highly unlikely given its unusual structure and unique genetic signature [42] ) or echinoderm diversification was extremely rapid. Taking the origin of stereom at around 525 Ma and the date of the earliest diversified faunas at between 515–510 Ma, the radiation of echinoderms into these fundamental body plans took place over a surprisingly short interval of just 10–15 my. Specimen collection and preparation Fieldwork was carried out during March and October 2012. After a preliminary survey of Lower–Middle Cambrian outcrops, five key sections were selected for more detailed investigation, the successions logged and the faunas collected. Articulated echinoderms were found to be restricted to specific horizons, which were often being commercially quarried for their articulated trilobite faunas. Fossils are preserved as moulds in shales and were studied by casting in latex and then whitening the latex with ammonium chloride sublimate before photography. How to cite this article: Smith, A.B. et al . The oldest echinoderm faunas from Gondwana show echinoderm body plan diversification was rapid. Nat. Commun. 4:1385 doi: 10.1038/ncomms2391 (2013).